Oncogenic gene expression and epigenetic remodeling of cis-regulatory elements in ASXL1-mutant chronic myelomonocytic leukemia Myeloid neoplasms are clonal hematopoietic stem cell disorders driven by the sequential acquisition of recurrent genetic lesions. Truncating mutations in the chromatin remodeler ASXL1 (ASXL1 MT ) are associated with a high-risk disease phenotype with increased proliferation, epigenetic therapeutic resistance, and poor survival outcomes. We performed a multi-omics interrogation to define gene expression and chromatin remodeling associated with ASXL1 MT in chronic myelomonocytic leukemia (CMML). ASXL1 MT are associated with a loss of repressive histone methylation and increase in permissive histone methylation and acetylation in promoter regions. ASXL1 MT are further associated with de novo accessibility of distal enhancers binding ETS transcription factors, targeting important leukemogenic driver genes. Chromatin remodeling of promoters and enhancers is strongly associated with gene expression and heterogenous among overexpressed genes. These results provide a comprehensive map of the transcriptome and chromatin landscape of ASXL1 MT CMML, forming an important framework for the development of novel therapeutic strategies targeting oncogenic cis interactions. Chronic myeloid neoplasms are malignant clonal hematopoietic stem cell disorders driven by recurrent genetic events, with an inherent risk of transformation to acute myeloid leukemia (AML) [1] , [2] . Within myeloid neoplasms, chronic myelomonocytic leukemia (CMML) represents an attractive disease model since it is characterized by both myelodysplastic and myeloproliferative features, while retaining a relatively simple clonal composition [3] . CMML shares the typical repertoire of genetic driver lesions with other myeloid neoplasms and is particularly enriched in truncating mutations involving ASXL1 (prevalence ~40%) [3] . The presence of truncating ASXL1 mutations in CMML is associated with proliferative disease features, resistance to epigenetic therapies, and adverse outcomes [4] , [5] , [6] . Due to their independent prognostic significance, ASXL1 mutations have been incorporated in all three contemporary molecularly integrated CMML-specific prognostic models [5] , [7] , [8] . Given the paucity of effective therapies for CMML, delineating the molecular mechanisms of ASXL1 -mutant CMML (ASXL1 MT ) is of particular interest from a therapeutic standpoint. The sum of evidence from mechanistic studies suggests that ASXL1 has a complex interactome, that truncating ASXL1 mutations promote leukemogenesis by transcriptional up-regulation of leukemogenic drivers including posterior HOXA genes, and that these mutations recruit several effectors to alter the epigenome through histone modifications, increases in chromatin accessibility, and remodeling of enhancers [9] , [10] , [11] , [12] , [13] , [14] . However, to our knowledge, no studies have been able to extensively query the epigenome in primary patient samples. Given the complexity of human transcriptional regulation in vivo and the multitude of potential epigenetic mechanisms cooperating to regulate transcriptional activity, questions remain about the interplay of regulatory mechanisms in patients with CMML. To elucidate this interplay, we interrogated the genome, transcriptome, and epigenome of patients with ASXL1 -wildtype (ASXL1 WT ) and ASXL1 MT CMML. In this work, we integrated somatic mutations, transcription, (hydroxy)methylation, histone modifications, and chromatin accessibility to reveal the complexity of the epigenetic landscape, the simultaneous presence of multiple regulatory mechanisms affecting drivers of leukemogenesis, and remodeling of the enhancer landscape as an important driver of intratumoral heterogeneity. These insights into the epigenetic landscape of ASXL1 MT CMML generated from primary patient samples are of considerable interest for the development of novel targeted therapeutic strategies for patients with ASXL1 MT CMML. To survey the epigenetic landscape of human CMML, we interrogated mutational spectrum, transcription, DNA methylation, histone modifications, and chromatin accessibility in ASXL1 MT ( n = 8) and ASXL1 WT ( n = 8) CMML (Fig. 1a ). 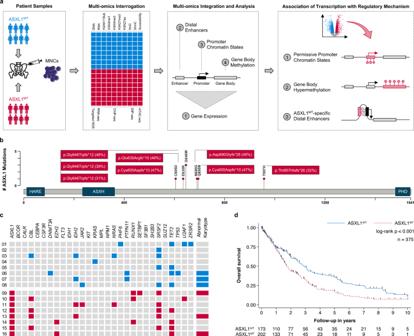Fig. 1: TruncatingASXL1mutations are of prognostic significance in chronic myelomonocytic leukemia and frequently co-occur with other mutations. aFlowchart showing the study design: An integrated multi-omics approach to discover ASXL1MT-specific epigenetic regulatory mechanisms associated with transcriptional up-regulation.bLollipop plot showing that all mutations inASXL1resulted in a frameshift preserving the HB1, ASXL, restriction endonuclease helix-turn-helix (HARE) and LXXLL motif alpha helical (ASXH) domain but not the plant homeodomain (PHD). All observed variant allele frequencies were compatible with heterozygosity.cHeatmap showing the spectrum of co-mutations, which included spliceosome components, chromatin regulators, modulators of DNA methylation, and cell signaling molecules. The prevalence of abnormal karyotypes and the burden of co-mutations were similar between ASXL1MTand ASXL1WTpatients.dKaplan–Meier plot showing overall survival estimates for the 375 patients with chronic myelomonocytic leukemia from which the 16 patients in this study were sampled from (median follow-up 18 months). The presence of truncatingASXL1mutations was associated with increased all-cause mortality in this patient population (median overall survival 1.72 years, 95% CI 1.51–2.19,n= 202 versus 2.92 years, 95% CI 2.39–3.61,n= 173; HR 1.54, 95% CI 1.19–1.98,p= 0.001). This association remained consistent after adjusting for age at diagnosis, sex, and the other factors of the Mayo Molecular Risk Stratification Model (HR 1.37, 95% CI 1.05–1.78,p= 0.019,n= 375)8. There were no violations of the proportional hazards assumption (p= 0.113). Source data are provided as a Source Data file. The clinical characteristics of the 16 patients with WHO-defined CMML included in this study are shown in Table 1 and Supplementary Data 2 . All mutations in ASXL1 resulted in a frameshift and were predicted to lead to a truncation of the protein’s plant homeodomain (Fig. 1b ). The spectrum of co-mutations was consistent with previous observations and included spliceosome components, chromatin regulators, modulators of DNA methylation, and cell signaling molecules (Fig. 1c ). Abnormal karyotypes were observed in the same number of patients and the burden of co-mutations was similar between the two groups (median number per group 3 versus 3, p = 0.508). This included several modulators of DNA methylation including TET2 , DNMT3A , and IDH2 (median number per group 1 versus 1, p = 0.699). As previously reported, G646W (c.1934dup) was the most prevalent ASXL1 mutation and the observed variant allele frequencies of all ASXL1 mutations were consistent with heterozygosity [15] , [16] . The presence of truncating ASXL1 mutations was associated with increased all-cause mortality in the larger patient population seen at our institution ( n = 375) from which the 16 patients is this study were sampled (Fig. 1d , Supplementary Fig. 1a, b ). For additional information on patient, sample, and cell selection, please refer to Methods and Supplementary Fig. 1c . Fig. 1: Truncating ASXL1 mutations are of prognostic significance in chronic myelomonocytic leukemia and frequently co-occur with other mutations. a Flowchart showing the study design: An integrated multi-omics approach to discover ASXL1 MT -specific epigenetic regulatory mechanisms associated with transcriptional up-regulation. b Lollipop plot showing that all mutations in ASXL1 resulted in a frameshift preserving the HB1, ASXL, restriction endonuclease helix-turn-helix (HARE) and LXXLL motif alpha helical (ASXH) domain but not the plant homeodomain (PHD). All observed variant allele frequencies were compatible with heterozygosity. c Heatmap showing the spectrum of co-mutations, which included spliceosome components, chromatin regulators, modulators of DNA methylation, and cell signaling molecules. The prevalence of abnormal karyotypes and the burden of co-mutations were similar between ASXL1 MT and ASXL1 WT patients. d Kaplan–Meier plot showing overall survival estimates for the 375 patients with chronic myelomonocytic leukemia from which the 16 patients in this study were sampled from (median follow-up 18 months). The presence of truncating ASXL1 mutations was associated with increased all-cause mortality in this patient population (median overall survival 1.72 years, 95% CI 1.51–2.19, n = 202 versus 2.92 years, 95% CI 2.39–3.61, n = 173; HR 1.54, 95% CI 1.19–1.98, p = 0.001). This association remained consistent after adjusting for age at diagnosis, sex, and the other factors of the Mayo Molecular Risk Stratification Model (HR 1.37, 95% CI 1.05–1.78, p = 0.019, n = 375) [8] . 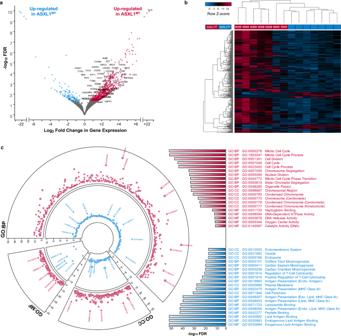Fig. 2: The transcriptome of ASXL1MTCMML is characterized by transcriptional up-regulation of key mitotic pathways and leukemogenic driver genes. aVolcano plot showing a predominance of transcriptional up-regulation in ASXL1MTCMML with a limited number of genes being down-regulated. Up-regulated therapeutic targets with therapeutic agents either being available or currently under development are labeled. Also labeled are the members of the posteriorHOXAcluster including the leukemogenic driverHOXA9and its co-factorMEIS1(bold).bHeatmap showing the separation of ASXL1MTand ASXL1WTCMML by unsupervised hierarchical clustering of all differentially expressed genes with FDR < 0.010.cCircos plot showing the up-regulation of mitotic activity and down-regulation of MHC class I mediated antigen presentation and cytotoxic T-cell activity in ASXL1MTCMML (red: up-regulated in ASXLMTCMML, blue: up-regulated in ASXLWTCMML). Bar graph showing the top hits in each gene ontology category (GO: Gene Ontology; BP: Biological Process; MF: Molecular Function; CC: Cellular Compartment). Axes represent the statistical significance of the gene ontology terms and the size of the markers is proportional to the number of genes per cluster. There were no violations of the proportional hazards assumption ( p = 0.113). Source data are provided as a Source Data file. Full size image Table 1 Clinical characteristics of 16 patients with CMML stratified by ASXL1 genotype. Full size table Truncating ASXL1 mutations are associated with transcriptional up-regulation of genes involved in cell cycle progression and DNA replication To define the gene expression profile associated with truncating ASXL1 mutations, we performed differential gene expression analysis (829 differentially expressed genes, FDR < 0.050, Fig. 2a , Supplementary Data 3 , Supplementary Fig. 2a–c ). There was a predominant up-regulation of transcriptional activity (707 genes) among ASXL1 MT patients. Of the 707 up-regulated genes in ASXL1 MT CMML, 217 were considered therapeutic targets (Fig. 2a , Supplementary Data 4 ) [17] . Unsupervised hierarchical clustering separated ASXL1 MT from ASXL1 WT patients (Fig. 2b ). Unlike previously reported, we did observe heterogeneous gene expression profiles among the non-G646W ASXL1 mutations [16] . The two ASXL1 MT patients with the most distally truncating mutations (Q695N and T957H) showed gene expression profiles intermediate between G646W and ASXL1 WT patients (Fig. 2b ). We had a priori classified the samples based on the genotype (ASXL1 MT versus ASXL1 WT ). Both samples in question clustered with the other ASXL1 MT samples with regards to their epigenetic features despite the apparent differences in their gene expression profiles (Supplementary Fig. 2d ). We therefore maintained our a priori sample classification based on the genotype (ASXL1 MT versus ASXL1 WT ) for all subsequent analyses. Functional annotation of the differentially expressed genes revealed several affected cellular processes including up-regulation of cell division (Supplementary Fig. 2e ) and down-regulation of MHC class I dependent antigen presentation (Fig. 2c ). Pathway analysis demonstrated an over-representation of genes involved in cell cycle (e.g. CDK1 , CCNA2 , CCNB2 ), DNA replication and repair (e.g. MCM10 , CDC6 , CDC45 ), gene expression (e.g. CHEK1 , RRM2 , BRCA1 ), signal transduction (e.g. HLA-A , VCAM1 , HLA-DQB1 ), and antigen presentation (e.g. CTSE , HLA-A , HLA-DQB1 ) pathways (Supplementary Fig. 2f , Supplementary Data 5 , 6 ). Fig. 2: The transcriptome of ASXL1 MT CMML is characterized by transcriptional up-regulation of key mitotic pathways and leukemogenic driver genes. a Volcano plot showing a predominance of transcriptional up-regulation in ASXL1 MT CMML with a limited number of genes being down-regulated. Up-regulated therapeutic targets with therapeutic agents either being available or currently under development are labeled. Also labeled are the members of the posterior HOXA cluster including the leukemogenic driver HOXA9 and its co-factor MEIS1 (bold). b Heatmap showing the separation of ASXL1 MT and ASXL1 WT CMML by unsupervised hierarchical clustering of all differentially expressed genes with FDR < 0.010. c Circos plot showing the up-regulation of mitotic activity and down-regulation of MHC class I mediated antigen presentation and cytotoxic T-cell activity in ASXL1 MT CMML (red: up-regulated in ASXL MT CMML, blue: up-regulated in ASXL WT CMML). Bar graph showing the top hits in each gene ontology category (GO: Gene Ontology; BP: Biological Process; MF: Molecular Function; CC: Cellular Compartment). Axes represent the statistical significance of the gene ontology terms and the size of the markers is proportional to the number of genes per cluster. Full size image Truncating ASXL1 mutations are associated with permissive promoter chromatin states supporting transcriptional up-regulation To understand the chromatin states associated with ASXL1 mutations, we integrated data on histone modifications (H3K4me1, H3K4me3, H3K27ac, and H3K27me3 ChIP-seq) and chromatin accessibility (ATAC-seq) by fitting a 7-state hidden Markov model (Fig. 3a ) [18] . First, we contrasted the two genotypes by subtracting the ASXL1 WT from the ASXL1 MT chromatin states. This genome-wide analysis revealed a transition of poised promoters and promoters with isolated chromatin accessibility to active promoters (loss of state 01 and 04, gain of state 05). This transition was mainly driven by H3K27ac and H3K4me1 gains in promoter regions. To verify that changes in promoter occupancy by the discovered chromatin states could serve as a plausible explanation for the observed transcriptional activity, we tested the associations between the presence of chromatin states and gene expression in ASXL1 MT CMML. As expected, the presence of active chromatin states was associated with increased gene expression (Fig. 3b ). Conversely, the presence of poised and repressed chromatin states was associated with decreased gene expression. There was a dosage effect with greater promoter region occupancy of a given state being associated with a greater magnitude of this effect in the expected direction (Fig. 3c ). Based on this model, promoter chromatin state transitions may serve as a plausible explanation for the observed changes in gene expression in ASXL1 MT CMML. Since the majority of the genes included in this genome-wide analysis were not expressed at all or not differentially expressed between the two genotypes, we performed a stratified analysis for the 707 up-regulated and 122 down-regulated genes in the ASXL1 MT patients identified by differential gene expression analysis (Fig. 3d ). Among the down-regulated genes there were chromatin state transitions between ASXL1 MT and ASXL1 WT CMML involving a loss of poised chromatin (01) and chromatin with isolated accessibility (04) towards both active (05) and repressed states (02). Among the up-regulated genes there was a marked increase of the active promoter state (05) around the transcription start site and losses of active chromatin states (05, 06) in the flanking regions. We did observe a gain in active chromatin states and / or loss of poised and repressed chromatin states in the promoter regions of the majority of up-regulated genes including mitotic kinases and several HOXA cluster genes (Fig. 3e ). However, for some genes (particularly two groups of relatively lowly expressed genes) we did not observe marked changes in promoter chromatin states between ASXL1 WT and ASXL1 MT CMML. 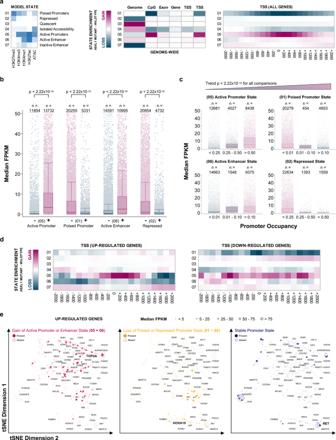Fig. 3: ASXL1MTCMML is associated with permissive promoter chromatin states supporting transcriptional up-regulation. aHeatmaps showing the chromatin states discovered by hidden Markov modeling and the transition of chromatin states between ASXL1WTand ASXL1MTCMML.bBox and strip plots showing the association between the presence of a given chromatin promoter state and gene expression (transcriptome-wide) among patients with ASXL1MTCMML (two-sided Mann–Whitney U test, rawp-values without adjustment for multiple hypothesis testing shown).cBox and strip plots showing the association between the extent of promoter occupancy of a given chromatin state and gene expression (transcriptome-wide) among patients with ASXL1MTCMML (two-sided Cuzick’s test for trend, rawp-values without adjustment for multiple hypothesis testing shown). The associations shown inbandcvalidate the model’s ability to predict gene expression and suggest that the transitions of these chromatin states between ASXL1WTand ASXL1MTCMML may serve as a plausible explanation for the observed differences in gene expression.dHeatmaps showing the chromatin state transitions in promoter regions between ASXL1WTand ASXL1MTCMML for the up- (n= 707) and down-regulated (n= 122) genes separately.eScatter plots showing the 707 up-regulated genes in two-dimensional tSNE space, clustered based on their promoter chromatin states. Color coding indicates the type of promoter chromatin state transition affecting each gene between ASXL1WTand ASXL1MTCMML. Marker size indicates the median gene expression among patients with ASXL1MTCMML. TheHOXAgenes,MEIS1, and the mitotic kinases are labeled. One representative gene from each group of promoter chromatin state transitions is highlighted (bold print) and corresponding ChIP-seq signal tracks are shown in Supplementary Fig.3e. Data are presented as standard Tukey boxplots (with the box encompassing Q1 to Q3, the median denoted as a central horizontal line in the box, and the whiskers covering the data within ±1.5 IQR in3bandc). Signal tracks for select up-regulated genes are shown in Supplementary Figure 3e . Importantly, some of the chromatin state transitions observed among the up-regulated genes (Fig. 3e ) were not obvious when performing the genome-wide analysis (Fig. 3a ). Consistent with previous observations, 5mC and 5hmC occupancy did not change significantly in the promoter regions of the differentially expressed genes (Supplementary Fig. 3a–d ) [19] . These data support the notion that promoter chromatin state transitions between ASXL1 WT and ASXL1 MT CMML are a plausible explanation for the up-regulation of gene expression in ASXL1 MT CMML. On average, the transition from inactive to active promoter chromatin states is strongly associated with increased transcriptional activity, but considerable heterogeneity exists among the up-regulated genes. Fig. 3: ASXL1 MT CMML is associated with permissive promoter chromatin states supporting transcriptional up-regulation. a Heatmaps showing the chromatin states discovered by hidden Markov modeling and the transition of chromatin states between ASXL1 WT and ASXL1 MT CMML. b Box and strip plots showing the association between the presence of a given chromatin promoter state and gene expression (transcriptome-wide) among patients with ASXL1 MT CMML (two-sided Mann–Whitney U test, raw p -values without adjustment for multiple hypothesis testing shown). c Box and strip plots showing the association between the extent of promoter occupancy of a given chromatin state and gene expression (transcriptome-wide) among patients with ASXL1 MT CMML (two-sided Cuzick’s test for trend, raw p -values without adjustment for multiple hypothesis testing shown). The associations shown in b and c validate the model’s ability to predict gene expression and suggest that the transitions of these chromatin states between ASXL1 WT and ASXL1 MT CMML may serve as a plausible explanation for the observed differences in gene expression. d Heatmaps showing the chromatin state transitions in promoter regions between ASXL1 WT and ASXL1 MT CMML for the up- ( n = 707) and down-regulated ( n = 122) genes separately. e Scatter plots showing the 707 up-regulated genes in two-dimensional tSNE space, clustered based on their promoter chromatin states. Color coding indicates the type of promoter chromatin state transition affecting each gene between ASXL1 WT and ASXL1 MT CMML. Marker size indicates the median gene expression among patients with ASXL1 MT CMML. The HOXA genes, MEIS1 , and the mitotic kinases are labeled. One representative gene from each group of promoter chromatin state transitions is highlighted (bold print) and corresponding ChIP-seq signal tracks are shown in Supplementary Fig. 3e . Data are presented as standard Tukey boxplots (with the box encompassing Q1 to Q3, the median denoted as a central horizontal line in the box, and the whiskers covering the data within ±1.5 IQR in 3b and c ). Full size image Transcriptional up-regulation in ASXL1 MT CMML is independent of gene body (hydroxy)methylation Given this heterogeneity of promoter chromatin states across the up-regulated genes, we sought to interrogate potential alternative epigenetic regulatory mechanisms that may explain the observed transcriptional activity. Aberrant genome-wide DNA methylation is associated with adverse cytogenetics features, increased leukemic transformation rates, and inferior survival outcomes in CMML [20] . However, differential DNA methylation in CMML is known to predominantly affect hematopoiesis-specific enhancers rather than promoter regions and gene bodies [19] , [21] . Not having observed differences in (hydroxy)methylation of promoter regions of the up-regulated genes (Supplementary Fig. 3a–d ), we interrogated gene body (hydroxy)methylation next. Gene body methylation was strongly associated with increased transcriptional activity (Fig. 4a ). However, there was no differential gene body methylation between ASXL1 WT and ASXL1 MT CMML for either the up- (Fig. 4b ) or down-regulated genes (Fig. 4c ). Similarly, gene body hydroxymethylation was strongly associated with increased transcriptional activity (Fig. 4d ). Again, there was no differential gene body hydroxymethylation between ASXL1 WT and ASXL1 MT CMML for either the up- (Fig. 4e ) or down-regulated genes (Fig. 4f ). In addition to the lack of differential (hydroxy)methylation in these stratified analyses, the co-mutations that might affect DNA (hydroxy)methylation were relatively balanced between the two ASXL1 genotypes (Fig. 1c ). 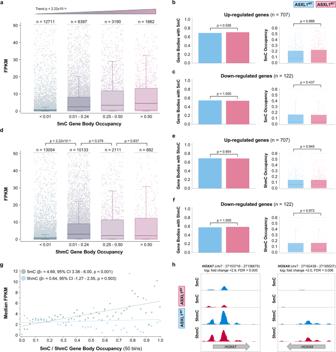Fig. 4: Gene body (hydroxy-)methylation is positively associated with gene expression but cannot serve as an explanation for the increased transcriptional activity given the lack of differential (hydroxy-)methylation betweenASXL1genotypes. aBox and strip plots showing the association between the extent of gene body methylation and gene expression (transcriptome-wide) among patients with ASXL1MTCMML (two-sided Cuzick’s test for trend, raw p-values without adjustment for multiple hypothesis testing shown).bBar graphs showing the lack of differential gene body methylation between ASXL1WTand ASXL1MTCMML for the up-regulated genes.cBar graphs showing the lack of differential gene body methylation betweenASXL1WTand ASXL1MTCMML for the down-regulated genes.dBox and strip plots showing the association between the extent of gene body hydroxymethylation and gene expression (transcriptome-wide) among patients with ASXL1MTCMML.eBar graphs showing the lack of differential gene body hydroxymethylation between ASXL1WTand ASXL1MTCMML for the up-regulated genes.fBar graphs showing the lack of differential gene body hydroxymethylation between ASXL1WTand ASXL1MTCMML for the down-regulated genes.gScatter plot showing the association between the extent of gene body (hydroxy)methylation and gene expression among patients with ASXL1MTCMML. Gene expression increases linearly with increases in gene body methylation. While the presence (compared to the absence) of gene body hydroxymethylation is strongly associated with increased gene expression, a greater extent of gene body hydroxymethylation is not associated with further increases in gene expression (threshold). The two-sided Wald test was used to test the model coefficients (raw p-values without adjustment for multiple hypothesis testing are shown).hSignal tracks showing the lack of differential (hydroxy-)methylation between ASXL1WTand ASXL1MTCMML for the up-regulated genesHOXA7andHOXA9. Data are presented as mean values (bars in4b,c,e,f) or standard Tukey boxplots (with the box encompassing Q1 to Q3, the median denoted as a central horizontal line in the box, and the whiskers covering the data within ±1.5 IQR in4a–f). The two-sided Mann–Whitney U test was used to compare groups in4b–f, rawp-values without adjustment for multiple hypothesis testing are shown. To ensure that the presence of TET2 , DNMT3A , or IDH2 co-mutations did not confound the (hydroxy)methylation status, we performed a stratified analysis that demonstrated no significant difference in global DNA (hydroxy)methylation (Supplementary Figure 4a ). We further validated these results using methylation microarrays (Supplementary Fig. 4b, c ). While transcriptional activity increased both in the presence of gene body methylation and hydroxymethylation, the effects of the extent of methylation and hydroxymethylation on gene expression were different. While a greater extent of gene body methylation was associated with increased transcriptional activity (dosage effect), there was no such relationship for hydroxymethylation (threshold effect, Fig. 4g ). Representative signal tracks for select genes of interest are shown in Fig. 4h . As an alternative unbiased approach, we identified 1595 differentially methylated regions (DMR, regions with FDR < 0.05) in the validation data set (microarray data). We mapped all hypermethylated regions to gene bodies requiring that there was no concurrent hypermethylation of the promoter region of the same gene. With this approach we identified one of the 707 up-regulated single genes (0.14%) with evidence of isolated gene body hypermethylation ( HBZ , log 2 -fold change in gene expression 4.25, FDR = 0.0008, DMR area=1.61, DMR FDR = 0.018). These data support the notion that gene body (hydroxy)methylation is associated with increased gene expression. However, the lack of differential (hydroxy)methylation between ASXL1 WT and ASXL1 MT for the up-regulated genes make it an unlikely explanation for the observed increase in transcriptional activity. Fig. 4: Gene body (hydroxy-)methylation is positively associated with gene expression but cannot serve as an explanation for the increased transcriptional activity given the lack of differential (hydroxy-)methylation between ASXL1 genotypes. a Box and strip plots showing the association between the extent of gene body methylation and gene expression (transcriptome-wide) among patients with ASXL1 MT CMML (two-sided Cuzick’s test for trend, raw p-values without adjustment for multiple hypothesis testing shown). b Bar graphs showing the lack of differential gene body methylation between ASXL1 WT and ASXL1 MT CMML for the up-regulated genes. c Bar graphs showing the lack of differential gene body methylation between ASXL1 WT and ASXL1 MT CMML for the down-regulated genes. d Box and strip plots showing the association between the extent of gene body hydroxymethylation and gene expression (transcriptome-wide) among patients with ASXL1 MT CMML. e Bar graphs showing the lack of differential gene body hydroxymethylation between ASXL1 WT and ASXL1 MT CMML for the up-regulated genes. f Bar graphs showing the lack of differential gene body hydroxymethylation between ASXL1 WT and ASXL1 MT CMML for the down-regulated genes. g Scatter plot showing the association between the extent of gene body (hydroxy)methylation and gene expression among patients with ASXL1 MT CMML. Gene expression increases linearly with increases in gene body methylation. While the presence (compared to the absence) of gene body hydroxymethylation is strongly associated with increased gene expression, a greater extent of gene body hydroxymethylation is not associated with further increases in gene expression (threshold). The two-sided Wald test was used to test the model coefficients (raw p-values without adjustment for multiple hypothesis testing are shown). h Signal tracks showing the lack of differential (hydroxy-)methylation between ASXL1 WT and ASXL1 MT CMML for the up-regulated genes HOXA7 and HOXA9 . Data are presented as mean values (bars in 4b , c , e , f ) or standard Tukey boxplots (with the box encompassing Q1 to Q3, the median denoted as a central horizontal line in the box, and the whiskers covering the data within ±1.5 IQR in 4a – f ). The two-sided Mann–Whitney U test was used to compare groups in 4b – f , raw p -values without adjustment for multiple hypothesis testing are shown. Full size image ASXL1 MT -specific distal enhancers are independently associated with transcriptional activity Cis-regulatory elements are powerful regulators of transcription and frequently altered in myeloid neoplasms [22] . Enhancers have been associated with aberrant transcriptional activity and response to treatment in CMML [23] . We identified candidate cis-regulatory elements by integrating chromatin accessibility and histone acetylation data. To explain increased transcriptional activity among ASXL1 MT patients, we hypothesized that the responsible cis-regulatory elements would only be present in ASXL1 MT but not ASXL1 WT CMML (genotype-specific cis-regulatory elements). Regions with chromatin accessibility (ATAC-seq) which were concurrently marked by H3K27ac and unique to ASXL1 MT were considered candidate regions (Fig. 5a, b ). There was no evidence for increased de-ubiquitination of H2AK119 in proximity of these genomic regions (Supplementary Fig. 5a ). The vast majority of the identified regions (92%) were annotated in ENCODE, with 75% of these regions demonstrating a distal enhancer-like signature (Fig. 5c ) and 2% being known super-enhancers [24] , [25] , [26] , [27] . Motif discovery revealed that these regions were predicted to bind ETS family transcription factors (Fig. 5d ) [28] . Intersection with publicly available ChIP-seq data confirmed the presence of ETS family transcription factors in these ASXL1 MT -specific enhancer regions (Fig. 5e ) [29] . BRD4 was also among the top 20 enriched transcription factors (effect size 2.05, p < 2.22 × 10 −16 ) and this enrichment was slightly more pronounced in the super-enhancer regions (effect size 2.59, p = 0.005). To associate the enhancers with putative target genes, we used a neighboring gene approach incorporating proximity on the linear genome, experimentally determined regulatory domains, and localization within conserved topologically associating domains (TADs) [30] , [31] . We excluded candidate regions overlapping with promoter regions and focused on distal enhancers (91% of the identified regions). These 3214 ASXL1 MT -specific distal enhancers were implicated in 4981 cis-interactions with 3308 genes (Fig. 5f ). Among these 3308 genes were 97 of the 707 up-regulated genes, an overlap unlikely to have occurred by chance ( p = 2.22 × 10 −6 ). Among these 97 up-regulated target genes were MEIS1 and 17 mitotic kinases including CDK1 , CCNE1 , and CDC20 (significant enrichment of mitotic cell cycle process, GO:1903047, FDR = 0.011). By virtue of the applied selection algorithm (GREAT) and additional constraints (TADs), most ASXL1 MT -specific distal enhancers were localized between 5 and 200 kb of their associated target gene (Fig. 5g ). The presence of a distal enhancer was positively associated with the expression of its target gene without evidence for a dosage effect when more than one enhancer was associated with a target gene (Fig. 5h ). The effect of the presence of a distal enhancer on the expression of its target gene decreased with increasing distance on the linear genome (Fig. 5i ). The genes associated with these ASXL1 MT -specific distal enhancers were involved in oncogenic MAPK and receptor tyrosine kinase signaling (Fig. 5j ). To understand if the presence of these enhancers is independently associated with increased gene expression, we fit multivariable-adjusted linear regression models. Among patients with ASXL1 MT CMML, the presence of these distal enhancers was independently associated with increased gene expression (Supplementary Fig. 5b ). The magnitude of this effect (the presence of an ASXL1 MT -specific distal enhancer) was comparable to a 20% increase in active promoter chromatin states or in gene body methylation. A measure of the relative importance of the different epigenetic regulatory mechanisms is shown in Supplementary Fig. 5c . Relevant regression diagnostics for the model are shown in Supplementary Fig. 5d–f . These data support the notion that ASXL1 MT -specific distal enhancers are independently associated with increased oncogenic gene expression and their presence can serve as a plausible explanation for the observed increased transcriptional activity including the overexpression of mitotic kinases. Fig. 5: ASXL1 MT -specific distal enhancers are positively associated with gene expression of their putative target genes and can serve as a plausible explanation for the increased transcriptional activity in ASXL1 MT CMML. a Venn diagram showing the co-mapping of chromatin accessibility and H3K27ac to identify ASXL1 MT -specific cis-regulatory elements. b Signal curves and heatmaps showing the co-occurrence of DNA accessibility and H3K27ac in these ASXL1 MT -specific cis-regulatory elements. c Venn diagram and bar graphs demonstrating the identity of these ASXL1 MT -specific cis-regulatory elements (known enhancers, mostly distally located). d Position weight matrices generated from motif discovery show the over-representation of ETS transcription factors (top 5 enriched motifs) in the ASXL1 MT -specific distal enhancers. e Validation of the predicted ETS transcription factor enrichment in the ASXL1 MT -specific distal enhancers using publicly available human transcription factor ChIP-seq data. f Euler diagrams and bar graphs showing the association between the ASXL1 MT -specific distal enhancers and putative target genes within leukemia-specific topologically associating domains. g Bar graphs showing the distribution of the ASXL1 MT -specific distal enhancers by distance on the linear genome from the transcription start site of their putative target genes. h Box and strip plots demonstrating the association between the presence of distal enhancers and increased gene expression among patients with ASXL1 MT CMML (without evidence for a dosage effect of more than one distal enhancer). i Box and strip plots demonstrating the association between proximity of distal enhancer and putative target gene on the linear genome and increased gene expression of the putative target gene among patients with ASXL1 MT CMML. j Bar graphs showing the functional annotation of the putative target genes of the ASXL1 MT -specific distal enhancers including receptor tyrosine kinase, cytokine, and oncogenic MAPK signaling. Data are presented as standard Tukey boxplots (with the box encompassing Q1 to Q3, the median denoted as a central horizontal line in the box, and the whiskers covering the data within ±1.5 IQR in 5h and i ). Full size image ASXL1 MT CMML is characterized by increased intratumoral heterogeneity due to increased chromatin accessibility in transcription factor binding sites Having identified ETS family transcription factors predicted to bind the ASXL1 MT -specific distal enhancers in proximity to several of the up-regulated genes, we performed single-cell ATAC-seq on three patients with ASXL1 WT (6832 cells) and three patients with ASXL1 MT CMML (5360 cells) to validate our bulk ATAC-seq findings (Supplementary Fig. 6a–e ). 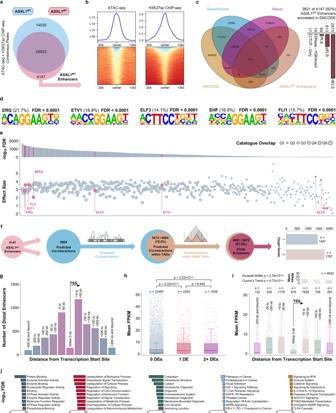Fig. 5: ASXL1MT-specific distal enhancers are positively associated with gene expression of their putative target genes and can serve as a plausible explanation for the increased transcriptional activity in ASXL1MTCMML. aVenn diagram showing the co-mapping of chromatin accessibility and H3K27ac to identify ASXL1MT-specific cis-regulatory elements.bSignal curves and heatmaps showing the co-occurrence of DNA accessibility and H3K27ac in these ASXL1MT-specific cis-regulatory elements.cVenn diagram and bar graphs demonstrating the identity of these ASXL1MT-specific cis-regulatory elements (known enhancers, mostly distally located).dPosition weight matrices generated from motif discovery show the over-representation of ETS transcription factors (top 5 enriched motifs) in the ASXL1MT-specific distal enhancers.eValidation of the predicted ETS transcription factor enrichment in the ASXL1MT-specific distal enhancers using publicly available human transcription factor ChIP-seq data.fEuler diagrams and bar graphs showing the association between the ASXL1MT-specific distal enhancers and putative target genes within leukemia-specific topologically associating domains.gBar graphs showing the distribution of the ASXL1MT-specific distal enhancers by distance on the linear genome from the transcription start site of their putative target genes.hBox and strip plots demonstrating the association between the presence of distal enhancers and increased gene expression among patients with ASXL1MTCMML (without evidence for a dosage effect of more than one distal enhancer).iBox and strip plots demonstrating the association between proximity of distal enhancer and putative target gene on the linear genome and increased gene expression of the putative target gene among patients with ASXL1MTCMML.jBar graphs showing the functional annotation of the putative target genes of the ASXL1MT-specific distal enhancers including receptor tyrosine kinase, cytokine, and oncogenic MAPK signaling. Data are presented as standard Tukey boxplots (with the box encompassing Q1 to Q3, the median denoted as a central horizontal line in the box, and the whiskers covering the data within ±1.5 IQR in5handi). 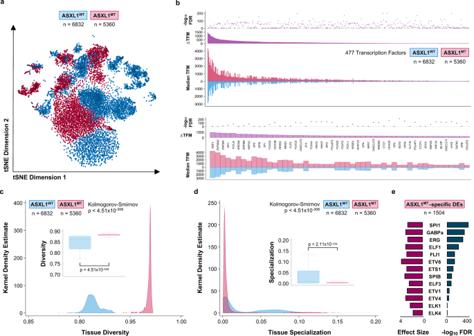Fig. 6: ASXL1MTCMML is associated with increased intratumoral heterogeneity secondary to an extended repertoire of accessible distal enhancers. aScatter plot showing 12192 single cells from CMML patients (stratified byASXL1genotype) in two-dimensional tSNE space, clustered based on the accessibility of known transcription factor motifs.bBar graphs and dot plot demonstrating the increased single-cell accessibility of binding sites for 476 transcription factors (top panel), ranked by the difference in accessible transcription factor motif (TFM) binding sites (scATAC-seq peaks with a given transcription factor motif) between ASXL1WTand ASXL1MTCMML. The top 50 transcription factors with increased accessible binding sites are magnified (bottom panel) and included key oncogenic myeloid transcription factors such as MZF1, MEF2C, and MEIS1. Source data are provided as a Source Data file.cArea graphs and box plots showing a measure of tissue diversity (based on single-cell entropies) for 12192 single cells from CMML patients (stratified byASXL1genotype). The two-sample Kolmogorov-Smirnov test for equality of distribution functions was used to compare both distributions. Source data are provided as a Source Data file.dArea graphs and box plots showing a measure of tissue specialization (based on single-cell entropies) for 12192 single cells from CMML patients (stratified byASXL1genotype). The two-sample Kolmogorov-Smirnov test for equality of distribution functions was used to compare both distributions (p-value). Source data are provided as a Source Data file.eBar graphs showing the enrichment of ETS transcription factor motifs in 1504 ASXL1MT-specific distal enhancers identified by scATAC-seq (validation of bulk ATAC-seq findings). Data are presented as standard Tukey boxplots (with the box encompassing Q1 to Q3, the median denoted as a central horizontal line in the box, and the whiskers covering the data within ±1.5 IQR in6candd). Cells from patients with ASXL1 MT CMML demonstrated increased chromatin accessibility as evidenced by an extended repertoire of accessible transcription factor motifs (Fig. 6b ). Among the top motifs were key oncogenic myeloid transcription factors including MZF1 (known to stimulate proliferation and delay differentiation), MEF2C (linked to therapeutic resistance), and MEIS1 (synergistic with HOXA9 in inducing leukemogenesis) [32] , [33] , [34] . We hypothesized that the increased chromatin accessibility could drive intratumoral heterogeneity in ASXL1 MT CMML. We calculated measures of tissue diversity and specialization for both genotypes and observed an increase in diversity with a reciprocal decrease in specialization in ASXL1 MT CMML (Fig. 6 c and d ). When examining 1504 ASXL1 MT -specific distal enhancers (identified by scATAC-seq), we again observed an enrichment of ETS family transcription factor motifs (Fig. 6e ). Similarly, BRD4 was again among the top 5 enriched transcription factors in these regions (effect size 2.32, p < 2.22 × 10 −16 ). These data support the notion that ASXL1 MT CMML is characterized by an increase in intratumoral heterogeneity with increased chromatin accessibility for transcription factors binding ASXL1 MT -specific distal enhancers. Fig. 6: ASXL1 MT CMML is associated with increased intratumoral heterogeneity secondary to an extended repertoire of accessible distal enhancers. a Scatter plot showing 12192 single cells from CMML patients (stratified by ASXL1 genotype) in two-dimensional tSNE space, clustered based on the accessibility of known transcription factor motifs. b Bar graphs and dot plot demonstrating the increased single-cell accessibility of binding sites for 476 transcription factors (top panel), ranked by the difference in accessible transcription factor motif (TFM) binding sites (scATAC-seq peaks with a given transcription factor motif) between ASXL1 WT and ASXL1 MT CMML. The top 50 transcription factors with increased accessible binding sites are magnified (bottom panel) and included key oncogenic myeloid transcription factors such as MZF1, MEF2C, and MEIS1. Source data are provided as a Source Data file. c Area graphs and box plots showing a measure of tissue diversity (based on single-cell entropies) for 12192 single cells from CMML patients (stratified by ASXL1 genotype). The two-sample Kolmogorov-Smirnov test for equality of distribution functions was used to compare both distributions. Source data are provided as a Source Data file. d Area graphs and box plots showing a measure of tissue specialization (based on single-cell entropies) for 12192 single cells from CMML patients (stratified by ASXL1 genotype). The two-sample Kolmogorov-Smirnov test for equality of distribution functions was used to compare both distributions ( p -value). Source data are provided as a Source Data file. e Bar graphs showing the enrichment of ETS transcription factor motifs in 1504 ASXL1 MT -specific distal enhancers identified by scATAC-seq (validation of bulk ATAC-seq findings). Data are presented as standard Tukey boxplots (with the box encompassing Q1 to Q3, the median denoted as a central horizontal line in the box, and the whiskers covering the data within ±1.5 IQR in 6c and d ). Full size image The gene expression profile of ASXL1 MT CMML is characterized by overexpression of proliferative genes, mirroring the clinical phenotype of leukocytosis, splenomegaly, resistance to epigenetic therapies (DNA methyltransferase inhibitors), and increased leukemic transformation rates [35] . Gaining a better understanding of the molecular mechanisms underlying this aberrant transcriptional activity is important for the development of novel therapies for patients with ASXL1 MT CMML. In this study we interrogated the epigenome of patients with ASXL1 MT CMML and observed a transition from poised and inactive to active chromatin states in promoter regions and increased chromatin accessibility exposing de novo distal enhancers correlating with the transcription of affected genes. We furthermore observed an increase in intratumoral heterogeneity due to an extended repertoire of transcription factor motifs, again involving ASXL1 MT -specific distal enhancers. These results suggest an important role of oncogenic cis interactions for the sustained expression of key drivers of leukemogenesis in ASXL MT CMML. The three ASXL proteins (ASXL1, ASXL2 and ASXL3) are mammalian homologs of Addition of sex combs (Asx) in Drosophila , a protein that regulates the balance of trithorax (activating) and polycomb (repressive) functions. In myeloid neoplasms, the ASXL1 gene is frequently affected by nonsense and frameshift mutations leading to truncation of the protein at the C-terminus and loss of the plant homeodomain (PHD) [15] . Hitherto, the associated proteins for the PHD of the Asx family remain unknown [36] . Investigations employing different disease models have shed light on the transcriptomic and epigenetic changes associated with ASXL1 loss and truncation. ASXL1 is thought to recruit chromatin modulators and transcription factors to alter transcriptional activity of genes involved in leukemogenesis. The exact molecular mechanisms associated with truncating ASXL1 mutations however remain to be defined. Based on the interaction between ASXL1 and BAP1, a predominant loss of polycomb repressive complex 1 (PRC1)-mediated histone de-ubiquitination was the initial expected mechanism regulating transcriptional activity in ASXL1 MT patients [12] , [37] . However, observations in ASXL1 MT AML cell lines suggested a predominant loss of polycomb repressive complex 2 (PRC2)-mediated histone methylation (loss of H3K27me3) to be the regulatory mechanism at work and implicated the deregulation of posterior HOXA cluster genes as key factors in the ensuing leukemogenesis [9] . Observations from an ASXL1 MT murine model suggested a gain of function of PRC1-mediated effects rather than altered PRC2 activity (unaffected H3K27me3) [13] . The notion that increased de-ubiquitination is facilitating the transcriptional up-regulation through enhanced activity of the ASXL1-BAP1 complex was further confirmed in different ASXL1 MT cell lines, however, a decrease in H3K27me3 was observed at the same time in this disease model [11] . Loss of both H3K27me3 and H2AK119Ub promoting the expression of leukemogenic posterior HOXA genes has since been confirmed in cell lines and a murine model [10] . Another ASXL1 MT murine model revealed an increase in chromatin accessibility along with the recruitment of the bromodomain and extra-terminal domain family member BRD4, resulting in enhanced expression of genes involved in stem-cell maintenance and myeloid differentiation [14] . Overall, the sum of evidence from these mechanistic studies suggests that ASXL1 has a complex interactome, that truncating ASXL1 mutations promote leukemogenesis by transcriptional up-regulation of leukemogenic drivers including posterior HOXA genes, and that these mutations recruit several effectors to alter the epigenome through histone modifications, increases in chromatin accessibility, and remodeling of enhancers [9] , [10] , [11] , [12] , [13] , [14] . Given the complexity of human transcriptional regulation in vivo and the multitude of potential epigenetic mechanisms cooperating to regulate transcriptional activity, we interrogated the genome, transcriptome, and epigenome of ASXL1 MT CMML using primary patient samples. Employing conservative statistical methods and relying on a robust number of biological replicates, we observed significant changes in promoter chromatin states and distal enhancers in ASXL1 MT CMML. In general, these changes were less extreme than the ones observed in data generated from different hematopoietic precursor and leukemic cell lines [9] , [11] . We interpret these differences as a consequence of greater biological variability in primary patient samples and the statistical framework employed in this study. While previous studies have focused on global changes in histone modifications and considered them in isolation, we integrated several omics layers using an unbiased machine learning approach to capture the complexity of the epigenetic landscape to a greater extent. In doing so, we observed significant differences between global trends in chromatin remodeling and changes affecting the differentially expressed genes of interest. This may indicate that global assessments of chromatin remodeling are only part of the information required to develop effective targeted epigenetic therapies for specific leukemogenic mechanisms. For many of the up-regulated genes, we observed chromatin state transitions towards active states driven by H3K27ac deposition in promoter regions. Similarly, we observed a loss of H2K27me3 affecting the promoter regions of several of the up-regulated genes (either in isolation or in concert with the aforementioned gains in active chromatin states). For several up-regulated, yet relatively lowly expressed genes the model did not reveal marked state transitions in the promoter regions. The global increase in the active promoter state also included gains in H3K4me1, which is of particular interest since KMT2A fusions, partial tandem duplications, abnormalities of KMT2C/KMT2D/SET1D/2D (COMPASS family) are exceedingly rare in CMML [38] . Another open question concerns the locus-specific effects of truncating ASXL1 mutations. While we observed widespread remodeling of the epigenome, we do not fully understand how truncated ASXL1 exerts its effects selectively across the epigenome. This represents a limitation of the current study and future work in suitable disease models may help further refine the list of targets of truncated ASXL1. While ChIP-seq studies with antibodies directed against truncated ASXL1 may reveal genomic loci of direct interaction, other ASXL1-mutant-specific effects may be mediated through protein-protein interactions [39] , [40] . Furthermore, our gene expression data did not support the gene expression profiles observed in different murine myeloid disease models (e.g. lack of HHEX up- and lack of SOX6 down-regulation in ASXL1 MT CMML) and it remains debatable how closely these models recapitulate human disease biology, given the inherent heterogeneity of human myeloid neoplasms [13] , [41] . In search of additional regulatory mechanisms for the up-regulated genes, we revisited promoter and gene body methylation without discovering compelling evidence for either mechanism being at work in ASXL1 MT CMML, despite the high prevalence of concurrent TET2 mutations [35] . This is consistent with previous observations in CMML pointing towards the importance of hematopoiesis-specific enhancers and may further be explained by the relatively balanced distribution of co-mutations in this study [19] , [21] . In CMML, aberrant methylation is known to be associated with distinct clinical features such as high-risk karyotypes and therapeutic resistance [20] , [23] . At the same time, the most commonly employed treatment strategy for CMML is the inhibition of DNMT with DNA methyltransferase inhibitors (i.e. azacytidine ± cedazuridine, decitabine), which are thought to epigenetically restore normal hematopoiesis in a subset of patients without altering the mutational burden or inherent risk of leukemic transformation [42] , [43] , [44] . Furthermore, subsequent translational investigations in CD14-selected peripheral blood mononuclear cells demonstrated that differential promoter methylation does not correlate with transcription in CMML [45] . Our DNA immunoprecipitation and microarray methylation studies using unselected bone marrow mononuclear cells do confirm these findings, so do our RNA-seq results in CD34-selected, CD14-selected, and unselected bone marrow mononuclear cells. Extending the search for plausible additional regulatory mechanisms, we discovered a group of distal enhancers with interesting characteristics. First, these enhancers were specific for ASXL1 MT CMML. Second, these enhancers associated with several of the genes up-regulated in ASXL1 MT CMML. Third, these enhancers tightly correlated with transcription independent of the prevalent promoter chromatin states and gene body (hydroxy)methylation. A model including promoter chromatin states, ASXL1 MT -specific distal enhancers, and gene body (hydroxy)methylation explained almost half of the variation in gene expression and adds to our understanding of the complexity of transcriptional regulation in ASXL1 MT CMML. These ASXL1 MT -specific distal enhancers were highly enriched in ETS family transcription factor motifs as well as BRD4 and explained part of the observed increase in intratumoral heterogeneity at the single-cell level. The mapping of these enhancers and their association with key up-regulated leukemogenic drivers such as MEIS1 and several mitotic kinases is of considerable interest given that the presence of such enhancers represents an explanation for the lineage- and context-specific transcriptional effects of novel therapeutic agents such as BET bromodomain inhibitors [46] , [47] . Observing BRD4 enrichment in the ASXL1 MT -specific distal (super-)enhancers, further support the exploration of these novel therapeutics for individualized treatment approaches in ASXL1 MT CMML. Here we drew a detailed map of oncogenic distal enhancers unique to a high-risk phenotype of CMML, laying the foundation for future mechanistic studies defining the viability of these aberrant cis interactions to serve as therapeutic targets. Genotype-specific oncogenic chromatin interactions may be exploited for therapeutic benefit and serve as the rationale for early phase clinical trials with emerging epigenetic small molecule therapeutics in a disease that has not seen significant therapeutic advances in the last 25 years [48] , [49] , [50] , [51] . Patient population, sample acquisition, and cell selection To survey the (epi-)genetic landscape of human CMML, we obtained bone marrow mononuclear cells from 16 patients with WHO-defined CMML (Table 1 ), half of which had truncating ASXL1 mutations. We performed targeted next generation sequencing of DNA, whole transcriptome RNA sequencing (RNA-seq), immunoprecipitation of DNA hydroxymethyl and methyl residues (DIP-seq), immunoprecipitation of the histone modifications H2AK119ub, H3K4me1, H3K4me3, H3K27ac, and H3K27me3 (ChIP-seq), and DNA transposase accessibility assays (ATAC-seq). The RNA-seq data were used to define the transcriptional activity in ASXL1 MT CMML and then correlated with known epigenetic regulatory mechanisms by integrating the ChIP-, DIP-, and ATAC-seq data. CMML is a malignant proliferation of monocytes and, unlike in acute myeloid leukemia, the fraction of CD34 + blasts is usually below 5% [35] . CD14 on the other hand is a marker of terminally differentiated monocytes as they appear in the peripheral blood and it is debatable whether the CD14 + cell population in the bone marrow represents the malignant cell population of interest in CMML. We refrained from further CD34- or CD14-sorting the bone marrow mononuclear cells for several reasons: First, the cell attrition rates due to CD34- and CD14-sorting would have made the multi-omics interrogation of primary patient samples for this study impossible (particularly the cell requirements for the ChIP-seq experiments). Second, we observed a tight correlation between the gene expression profiles of sorted and unsorted cells, raising the question whether cell sorting would have influenced the results significantly (Supplementary Fig. 2a–c ). Third, our methylation analysis on unsorted cells confirms the results generated from CD14-sorted monocytes [45] . Avoiding excessive cell attrition due to sorting, we have been able to perform all analyses with at least five biological replicates per group. There were 16 patients included in this study and we performed experiments on all available samples for these patients. Supplementary Fig. 1c shows the samples that were included in the analysis after performing sample and data quality control. There were 14 samples for RNA-seq (87.5%), 15 for H2AK119ub ChIP-seq (93.8%), 15 for H3K27ac ChIP-seq (93.8%), 12 for H3K27me3 (75.0%), 14 for H3K4me1 ChIP-seq (87.5%), 11 for H3K4me3 ChIP-seq (68.8%), 15 for 5mC DIP-seq (93.8%), 15 for 5hmC DIP-seq (93.8%), and 11 for ATAC-seq (68.8%). The 16 patients included in this study were sampled from a population of 576 patients with WHO-defined CMML seen at the Mayo Clinic in Rochester, Minnesota [52] . All studies were approved by the Mayo Clinic Institutional Review Board. Written informed consent was obtained from all patients in accordance with the Declaration of Helsinki. Bone marrow mononuclear cells were collected in EDTA tubes and selected using Ficoll-Hypaque density gradient centrifugation (Sigma-Aldrich, St. Louis, United States). Genomic DNA was isolated using the ACCEL-NGS 1 S Plus DNA Library Kit (Swift Biosciences, Ann Arbor, United States). Total RNA was analyzed by preparing cDNA libraries generated in accord with the RNA-seq preparation protocol (Illumina, San Diego, United States). Viable bone marrow mononuclear cells were stored in freezing medium (10% DMSO, 40% fetal bovine serum, 40% RPMI) at −80 °C. DNA targeted next-generation sequencing For 375 of the 576 patients complete clinical information as well as genetic information from a 36-gene panel targeted next-generation sequencing assay were available for prognostic modeling. The regions of these 36 genes were selected for custom target capture using Agilent SureSelect Target Enrichment Kit (Agilent Technologies, Santa Clara, United States). Libraries derived from each DNA sample were prepared using NEB Ultra II (New England Biolabs, Ipswitch, United States) and individually barcoded by dual indexing. Sequencing was performed on an HiSeq 4000 (Illumina) with 150 bp paired-end reads. Forty-eight pooled libraries per lane were sequenced to a median read depth of ~400x. The custom panel of target regions covered all coding regions and consensus splice sites from the following 36 genes: ASXL1 , CALR , CBL , CEBPA , DNMT3A , EZH2 , FLT3 , IDH1 , IDH2 , IKZF1 , JAK2 , KRAS , MPL , NPM1 , NRAS , PHF6 , PTPN11 , RUNX1 , SETBP1 , SF3B1 , SH2B3 , SRSF2 , TET2 , TP53 , U 2AF1 , and ZRSR2 . Paired-end reads were processed and analyzed as previously described [8] . RNA-seq and qPCR RNA quality was determined using an Agilent Bioanalyzer RNA Nanochip or Caliper RNA assay. Library preparation was performed using TruSeq Stranded Total RNA (Illumina) and sequenced on an HiSeq 2500 (Illumina) with paired-end reads. RNA-seq sequencing reads were processed through the MAPRSeq bioinformatics workflow as previously described [53] . Reads were aligned to the GRCh38 reference genome and transcript counts calculated using featureCounts (v2.0.0) [54] . Differential expression was performed using DESeq2 (v1.30.1), clustering using heatmap.2 (v3.1.1, https://CRAN.R-project.org/package=gplots ), and plotting using EnhancedVolcano (v1.8.0, https://github.com/kevinblighe/EnhancedVolcano ) [55] . Pathway analyses were performed using gProfiler (v2021-05-01) and the Reactome Pathway Knowledgebase (v2021-5-7) [56] , [57] . Potential therapeutic targets among the up-regulated genes were identified by querying DGIdb (v3.0) [17] . For the validation of RNA-seq results we analyzed a subset of target genes by quantitative Reverse Transcription Polymerase Chain Reaction (RT-qPCR). Total RNA from the RNA-seq experiments was used to synthetize cDNA with the High-Capacity cDNA Reverse Transcription Kit (Applied Biosystems, Carlsbad, United States). A 1/3 dilution of the total cDNA was amplified by real-time PCR. Samples were prepared with PerfeCTa SYBR Green FastMix (Quanta BioSciences, Gaithersburg, United States), the primer sets are given in Supplementary Data 1 . ChIP-seq Approximately 100,000 cells from each sample were used for input for native chromatin immunoprecipitation (N-ChIP). Cells were lysed on ice for 20 min in lysis buffer containing 0.1% Triton X-100, 0.1% deoxycholate, and protease inhibitor. Extracted chromatin was digested with 90U of MNase enzyme (New England Biolabs) for 6 min at 25 °C. The reaction was quenched with 250 µM of EDTA post-digestion. A mix of 1.0% Triton X-100 and 1.0% deoxycholate was added to the digested samples and incubated on ice for 20 min. Digested chromatin was pooled and pre-cleared in IP buffer (20 mM Tris-HCl [pH 7.5], 2 mM EDTA, 150 mM NaCl, 0.1% Triton X-100, and 0.1% deoxycholate) plus protease inhibitors with pre-washed Protein A/G Dynabeads (Thermo Fisher Scientific, Waltham, United States) at 4 °C for 1.5 h. Supernatants were removed from the beads and transferred to a 96-well plate containing the antibody-bead complex. Following an overnight 4 °C incubation, samples were washed twice with low salt buffer (20 mM Tris-HCl [pH 8.0], 0.1% SDS, 1.0% Triton X-100, 2 mM EDTA, and 150 mM NaCl) and twice with high salt buffer (20 mM Tris-HCl [pH 8.0], 0.1% SDS, 1.0% Triton X-100, 2 mM EDTA, and 500 mM NaCl). DNA-antibody complexes were eluted in elution buffer (100 mM NaHCO 3 , 1.0% SDS), incubated at 65 °C for 90 min. Protein digestion was performed on the eluted DNA samples at 50 °C for 30 min using protease mix (QIAGEN, Venlo, Netherlands). ChIP DNA was purified using Sera-Mag beads (Thermo Fisher Scientific) with 30% PEG before library construction. H2AK119ub and H3K27ac ChIP-seq was performed as previously described [58] . The antibodies were used at a dilution of 1:250 (H3K27me3), 1:500 (H3K4me1 and H3K4me3), and 1:1000 (H2AK119ub and H3K27ac). Libraries were prepared by following a modified Illumina paired-end protocol and sequenced on an HiSeq 2500 (Illumina) to a median depth of ~25 million (H3K4me1 and H3K4me3) or ~50 million reads (H3K27me3 and Input). Reads were aligned to the GRCh38 reference genome using bowtie2 (v2.3.3.1) [59] . DIP-seq and methylation microarrays Genomic DNA was isolated and submitted to the Mayo Clinic Epigenomics Development Laboratory (EDL) for DNA immunoprecipitation and library preparation. The 5mC-33D3 (C15200081) monoclonal antibody (Diagenode, Denville, United States), an in-house developed 5hmC antibody (EDL), and the 53017 bridging antibody (Active Motif, Carlsbad, United States) were used. The antibodies were used at a dilution of 1:110 (5hmC) and 1:340 (5mC). Libraries were prepared by following a modified Illumina paired-end protocol and sequenced on a HiSeq 4000 (Illumina). Reads were aligned to the GRCh38 reference genome using the Burrows-Wheeler Aligner [60] . For the validation of DIP-seq results we analyzed a subset of samples on the Infinium MethylationEPIC (850 K) array (Illumina) according to the manufacturer’s specifications. Signal intensities were processed and normalized using Minfi (v1.36.0) using subset within-array quantile normalization [61] , [62] . CpGs below the detection threshold ( p < 0.010) as well as unreliable and cross-reactive probes were removed, leaving 787403 CpGs for downstream analyses. Differentially methylated regions were identified using bumphunter (v1.32.0) [63] . ATAC-seq and single-cell ATAC-seq DNA for ATAC-seq was prepared from 50,000 cells following the OMNI-ATAC procedures as described by Corces et al. with modifications using the Nextera kit (Illumina) [64] . The cells were lysed for 3 min on ice and transposed for 30 min at 37 °C following clean-up. The DNA libraries were prepared with 5–10 cycles of PCR amplification with the NEB High Fidelity Master Mix (New England Biolabs, Ipswich, United States). Clean-up was done using the Zymo DNA Clean and Concentrator kit (Zymo Research, Irvine, United States) and followed with AMPure XP (Beckman Coulter, Brea, United States) bead clean-up to remove primer dimers and under-digested chromatin. Sequencing was performed on an HiSeq 4000 (Illumina) to a depth of ~30 million reads per sample. Reads were aligned to GRCh38 using bowtie2 [59] . For the single-cell chromatin transposase accessibility assays (scATAC-seq) cryopreserved bone marrow mononuclear cells were thawed and resuspended following an established workflow (thawing, resuspension, sequential dilution, centrifugation, straining, viability assessment) and approximately 100000 viable mononuclear cells per sample were subjected to transposase assays (exposing buffered nuclei to Tn5 transposase) before proceeding to single-cell partitioning into gel beads in emulsion, barcoding, library construction, and sequencing following established 10X Genomics protocols. The target cell recovery was approximately 2000 cells per sample. For details on the 10X Genomics Chromium platform including demonstrated protocols on sample preparation, library construction, instrument settings, and sequencing parameters please see the manufacturer’s resources ( https://support.10xgenomics.com/single-cell-atac ). Genomic libraries were sequenced on an HiSeq 4000 (Illumina) before demultiplexing, alignment to the reference genome, and post-alignment quality control. The 10X Genomics Cell Ranger ATAC software (v2.0) was used for demultiplexing, alignment of the reads to the GRCh38 reference genome, filtering and quality control, counting of barcodes and unique molecular identifiers, identification of transposase cut sites, detection of accessible chromatin peaks, count matrix generation for peaks and transcription factors. Consensus peak calling Aligned reads from the different immunoprecipitation and accessibility sequencing experiments were sorted and indexed using samtools (v1.9) and peaks were called using MACS2 (v3.0.0a6) with input controls (except ATAC-seq) [65] , [66] . Peak calling with default parameters was performed before subjecting the peaks to the MSPC (v5.4.0) consensus peak calling algorithm [67] . By convention H3K4me1, H2AK119ub, and H3K27me3 peaks were called as “broad peaks” and the remaining marks were called as “narrow peaks”. To leverage the power of several biological replicates per analysis we employed a standard peak calling threshold in MACS2 (FDR < 0.050) before applying a more stringent threshold in the subsequent MSPC step (weak threshold p < 1.00 × 10 −4 , stringency threshold p < 1.00 × 10 −8 ). The UCSC Genome Browser and deepTools (v3.5.0) were used for signal visualization [68] , [69] . For visualization purposes averaged, input-corrected average signal tracks were created (except ATAC-seq where no input was used) using wiggletools mean (v1.2) and deepTools bamCoverage / bigwigCompare [70] . Data analysis Data are presented as median (range) unless denoted otherwise. Medians were the preferred measure of central tendency and non-parametric hypothesis tests were used for comparisons unless stated otherwise. Continuous variables were compared using the Mann-Whitney-U test, categorical variable using Fischer’s exact test. Trends across ordered groups were assessed using Cuzick’s test for trend. The equality of single-cell entropy distributions was evaluated using the two-sample Kolmogorov-Smirnov test. Overall and leukemia-free survival estimates were calculated using the Kaplan and Meier method [71] . Overall survival was defined as the time from diagnosis to death and patients who were alive at the end of follow-up were censored. Leukemia-free survival was defined as the time from diagnosis to leukemic transformation or death and patients who were alive and free of acute leukemia at the end of follow-up were censored. The log-rank test was used to compare time to event data in subgroups. Multivariable-adjusted (Cox) proportional hazards regression models were used to assess the association between clinical and genetic parameters of interest and overall survival [72] . Violations of the proportional hazards assumption were evaluated using Schoenfeld residuals. Hidden Markov modeling (ChromHMM v1.22) was used to discover and characterize the presence of chromatin states in promoter regions (TSS ± 2000bp) [18] . We fit 5- to 15-state models and judged their goodness of fit by each model’s ability to discriminate important chromatin states (active promoter, poised promoter, active enhancer, inactive enhancer, repressed, quiescent) without creating an excessive number of combinatorial states within each epigenetic mark. Based on the ability to sufficiently discriminate the activity of promoters and enhancers, the 7-state model was felt to be the most parsimonious model with acceptable fit for the data. Candidate cis-regulatory elements were validated using the ENCODE, GeneHancer, and Hacer databases [24] , [25] , [27] . To annotate and associate these regions with potential target genes, the Genomic Regions Enrichment of Annotations Tool (GREAT v4.0.4) was used [30] . To increase the specificity of the predicted (enhancer-promoter) cis-interactions, we included only those that did not violate the boundaries of topologically associating domains established in K562 cells [31] . Super-enhancers were identified by intersecting the candidate cis-regulatory elements with known super-enhancers in K562 cells [26] . De novo motif analysis was performed using Hypergeometric Optimization of Motif EnRichment (HOMER v3.0) [28] . Candidate transcription factors predicted to bind these regions were then validated by querying the ReMap 2020 database [29] . To estimate the independent effect of each epigenetic regulatory mechanism on gene expression, we employed multivariable-adjusted linear regression. Given the heavily left-skewed distribution and overdispersion of transcript count data we performed a log-transformed of the transcript count data (adding a pseudocount). We then used ordinary least squares regression to model the transformed transcript count data and exponentiated the obtained regression coefficients for ease of interpretation of the effect sizes ( e β − 1). The model included the active and inactive chromatin states, gene body (hydroxy)methylation, and the presence of an associated distal enhancer as parameters. We used the lmg metric (hierarchical partitioning of R 2 ) as an estimate of relative importance for each model paramaters [73] , [74] . Routine regression diagnostics were employed to evaluate model assumptions and model fit (including assessments of influence, leverage, and multicollinearity). Observations with excessive leverage ( h > [(2 * k )/ n ]) and influence (Cook’s D > [4/( n − k − 1)]) were removed ( n denoting the sample size and k the number of model parameters). Quality control, integration, normalization (TF-IDF), scaling, feature selection, clustering, and dimensionality reduction (SVD) of the scATAC-seq data was performed using Seurat (v4.0.5) [75] . Batch correction was performed using Harmony (v0.1.0) [76] . Single-cell entropies were calculated using BioQC (v1.18.0) [77] , [78] . Reporting summary Further information on research design is available in the Nature Research Reporting Summary linked to this article.